Bacterial variability in the mammalian gut captured by a single-cell synthetic oscillator Synthetic gene oscillators have the potential to control timed functions
and periodic gene expression in engineered cells. Such oscillators have been refined
in bacteria in vitro, however, these systems have lacked the robustness and
precision necessary for applications in complex in vivo environments, such as the
mammalian gut. Here, we demonstrate the implementation of a synthetic oscillator
capable of keeping robust time in the mouse gut over periods of days. The
oscillations provide a marker of bacterial growth at a single-cell level enabling
quantification of bacterial dynamics in response to inflammation and underlying
variations in the gut microbiota. Our work directly detects increased bacterial
growth heterogeneity during disease and differences between spatial niches in the
gut, demonstrating the deployment of a precise engineered genetic oscillator in
real-life settings. Oscillators are extensively utilized as clocks and timers in computation
and biology [1] , [2] . Synthetic gene oscillators
in bacterial cells have been developed and refined over past
decades [3] , [4] , [5] , [6] , [7] , [8] , [9] , [10] , [11] , [12] , led by the development of the repressilator
circuit—a simple negative feedback loop constructed from three transcriptional
repressor proteins, which inhibit each other’s expression in turn (Tn10 TetR,
bacteriophage λ CI and Escherichia coli LacI) [3] . Engineered bacteria hold great promise for
deployment as diagnostics and therapeutics in the clinic [13] . Oscillatory gene control
could enable increasingly complex applications for engineered bacteria, for example
controlling time-linked functionality or sophisticated recorders and
counters. Differential bacterial growth underlies colonization of the gut by
commensal species during childhood, pathogenic infection, and the establishment of
dysbiosis in the microbiota that has been linked to an increasing array of
diseases [14] . Recently, several methods have been developed
to estimate instantaneous, average bacterial growth rates using metagenomic
sequencing data [15] , [16] , [17] , [18] . These methods have
provided insights into spatial and temporal changes in comparative growth
rate [19] , [20] . However,
single-cell methods offer different advantages, in particular providing valuable
information about growth variability across a population [21] , [22] , [23] , [24] , [25] , [26] , [27] , [28] , [29] . Such information is crucial to our
understanding of bacterial growth in the gut, which includes a broad range of niches
with different growth favorability for any given bacterial species, potentially
limiting the interpretation of average growth measures. Similarly, methods that can
quantify absolute, rather than relative, growth and that assess growth in
aggregate [21] , [30] , rather than
as instantaneous rates, are particularly important for developing a comprehensive
understanding of growth in a non-invasive manner. The original repressilator was recently redesigned to afford a highly
regular and robust oscillator with reduced error propagation and information losses,
referred to herein as the repressilator 2.0 (Fig. 1a ; Supplementary Fig. 1 ) [5] . During in vitro growth the circuit keeps phase
in single cells for hundreds of bacterial generations, with an oscillation period
that is growth-rate independent and linked to bacterial
divisions [5] . The circuit’s low variance between cells, and
independence from external feedback and entrainment cues make it an attractive timer
for use in complex environments. Fig. 1 RINGS analysis measures single-cell repressilator 2.0 phase. a The repressilator is a
ring-oscillator comprising three repressors. b Colonies expressing the repressilator 2.0 display
fluorescent rings controlled by the circuit’s oscillations. c Repressilator phase
progresses based on bacterial divisions, with an ~15 generation
period. The phase of the colony-initiating bacterium at the time of
plating ( θ 0 ) controls the position of
the fluorescent rings forming within that colony. d The RINGS pipeline consists of plating
of a bacterial population on agar plates, followed by imaging,
computational identification and export of individual, centered
colonies and fitting of a generative model. The fit of ring position
is then used to estimate θ 0 at the time of plating. e LPT239 bacteria, carrying the
repressilator, are synchronized by exposure to aTc or IPTG as
demonstrated by average projections of aligned colony images
compared to unsynchronized controls. Scale = 0.1 cm. e RINGS analysis demonstrates the ability
of the repressilator to report on bacterial phase. Graph shows polar
histogram representing normalized counts of colonies (radius) within
a given θ 0 range (angle). For e , f IPTG n = 93; aTc n = 62; unsync n = 49. g LPT320
bacteria were synchronized with aTc and grown in log-phase growth at
37 °C, plating samples for colony counts and RINGS analysis every
2 h ± 15 min. h RINGS analysis
measured phase ( θ 0 ) across the population. Graphs show histograms of normalized θ 0 count for two biological
replicates. Arrows indicate shift in population since last timepoint i . Repressilator phase
correlates with the estimated generations as determined by CFU
counts from agar plating. Graph shows mean with 95% CI (error bars
smaller than datapoints) of elapsed phase after removal of aTc. j Cumulative distribution
functions of predicted generations elapsed across the population. Labels list average generations for each timepoint as calculated by
CFU counts in panel i . For h – j , the number of colonies analyzed are listed in j . Source data are provided as
a Source Data file Full size image Here, we use the repressilator 2.0 to infer bacterial growth dynamics at
a single-cell level. We develop and validate an imaging analysis pipeline to
determine repressilator phase. In this way, we investigate bacterial population
dynamics during colonization of, and growth within, the mammalian gut. Our results
show increased growth variability under inflamed conditions, demonstrating the
importance of single-cell methods for reliable bacterial growth analysis. We also
reveal robust functionality and controllability of the repressilator 2.0 across
diverse host and environmental contexts. RINGS method development and testing Because bacterial colonies expand radially in a uniform manner, with
division only occurring at the periphery [31] , synchronous
repressilator 2.0 oscillations create stable macroscopic rings when fluorescent
reporters are driven under repressilator 2.0 control (Fig. 1b ) [5] . The phase of a bacterium that seeds a
colony determines the phase, and thus fluorescent reporter expression, of each
subsequent generation throughout the colony. As such, the positions (i.e.,
radii) of the fluorescent rings in a colony are indicative of the phase of the
bacterium that seeded the colony (Fig. 1c ). To utilize this behavior, we developed a workflow for bacterial
colony image capture and processing, which we call R epressilator-based IN ference of G rowth at S ingle-cell level (RINGS)
(Fig. 1d ). The process begins with
fluorescent macroscope imaging of repressilator 2.0-expressing bacterial
colonies. Image analysis then identifies colonies and fits a generative model to
the fluorescent rings within each colony. The ring positions are used to
estimate the relative phase of the single bacterium that seeded the colony at
the time of plating ( θ 0 ). Because repressilator 2.0
progression is linked to bacterial growth [5] , the elapsed phase
between two timepoints can be used to infer bacterial growth. Given the periodic
nature of the oscillator, meaning that the circuit’s output is the same in any
given period (i.e., values are modulo 2π), adjusting the sampling frequency to
ensure that less than a period elapses between timepoints allows unambiguous
determination of growth. 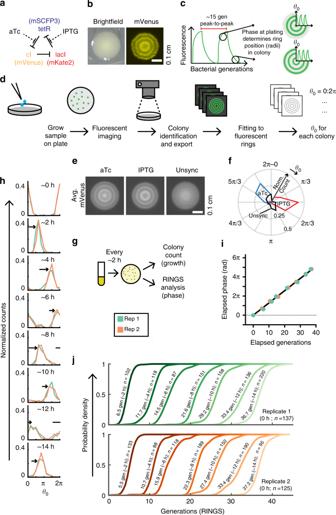Fig. 1 RINGS analysis measures single-cell repressilator 2.0 phase.aThe repressilator is a
ring-oscillator comprising three repressors.bColonies expressing the repressilator 2.0 display
fluorescent rings controlled by the circuit’s oscillations.cRepressilator phase
progresses based on bacterial divisions, with an ~15 generation
period. The phase of the colony-initiating bacterium at the time of
plating (θ0) controls the position of
the fluorescent rings forming within that colony.dThe RINGS pipeline consists of plating
of a bacterial population on agar plates, followed by imaging,
computational identification and export of individual, centered
colonies and fitting of a generative model. The fit of ring position
is then used to estimateθ0at the time of plating.eLPT239 bacteria, carrying the
repressilator, are synchronized by exposure to aTc or IPTG as
demonstrated by average projections of aligned colony images
compared to unsynchronized controls. Scale = 0.1 cm.eRINGS analysis demonstrates the ability
of the repressilator to report on bacterial phase. Graph shows polar
histogram representing normalized counts of colonies (radius) within
a givenθ0range (angle). Fore,fIPTGn= 93; aTcn= 62; unsyncn= 49.gLPT320
bacteria were synchronized with aTc and grown in log-phase growth at
37 °C, plating samples for colony counts and RINGS analysis every
2 h ± 15 min.hRINGS analysis
measured phase (θ0) across the population.
Graphs show histograms of normalizedθ0count for two biological
replicates. Arrows indicate shift in population since last timepointi. Repressilator phase
correlates with the estimated generations as determined by CFU
counts from agar plating. Graph shows mean with 95% CI (error bars
smaller than datapoints) of elapsed phase after removal of aTc.jCumulative distribution
functions of predicted generations elapsed across the population.
Labels list average generations for each timepoint as calculated by
CFU counts in paneli. Forh–j, the number of colonies analyzed are listed inj. Source data are provided as
a Source Data file E.coli LPT239 bacteria expressing
the repressilator 2.0 (Supplementary Table 1 ) were phase-synchronized by growth in the presence of
Isopropyl β-D-1-thiogalactopyranoside (IPTG) or anhydrotetracycline (aTc), which
interrupt repression by LacI and TetR, respectively (Fig. 1a ). Analysis of YFP fluorescence by colony
imaging (Fig. 1e ) and RINGS analysis
(Fig. 1f ) demonstrated the ability
for RINGS to distinguish between these two distinct oscillator phases. Further
optimization through variation of the ‘sponge plasmid’ (Supplementary
Fig. 1 ), a key element in previous
efforts to reduce oscillation variability in the repressilator 2.0
circuit [5] , yielded more consistent fluorescent rings
within colonies and allowed subsequent RINGS analyses using combined CFP and YFP
fluorescence data (Supplementary Fig. 2 ). To further test the ability of RINGS to track bacterial growth over
time, we sampled aTc-synchronized E. coli LPT320 bacteria (Supplementary Table 1 ), kept in constant log-phase culture by back-dilution and
plated at ~2-h intervals. Plates were imaged and analyzed using RINGS to measure
repressilator phase, and for colony forming unit (CFU) counts to measure average
bacterial growth (Fig. 1g ). Repressilator 2.0 phase progressed coherently according to bacterial growth of
the population (Fig. 1h, i ,
Supplementary Fig. 3a, b ), with
regression of the elapsed phase (RINGS) vs growth (CFU) data quantifying the
LPT320 repressilator 2.0 period length as 15.4 ± 0.2 SEM gen/period
(Fig. 1i ). This is consistent with
previous period measures of similar circuits [5] . The period length allows
assignment of a distribution of probable growth on a single-cell level, forming
a cumulative probability distribution for the population (Fig. 1j ). RINGS is robust to strain and environmental variations The repressilator was transferred to E.
coli (MG1655 - PAS715; and the human probiotic strain, Nissle
1917 – PAS717) and Salmonella
enterica serovar Typhimurium (hereafter referred to as S . Typhimurium) (LT2-PAS716) strains
(Fig. 2a–c ; Supplementary
Table 1 ), where RINGS again
faithfully tracked cell divisions (Fig. 2d–f ). The period of the repressilator was determined in each
case either using the regression of RINGS vs growth curves (Fig. 2d–f ) or during growth in a microfluidic device
capable of trapping cells for fluorescent microscopic analysis over multiple
repressilator cycles (Supplementary Fig. 4a,
b ; Table 1 ) [32] . Both methods quantified the same period
for E. coli PAS715 bacteria grown in rich
medium (RINGS: 15.3 ± 0.8 SEM gen/period; mother machine: 15.3 ± 0.2 SEM
gen/period) (Fig. 2d ; Table 1 ), with a similar period also calculated for S . Typhimurium PAS716 and E. coli Nissle 1917 PAS717 bacteria using RINGS
(PAS716: 16.4 ± 1.5 SEM gen/period; PAS717: 15.3 ± 1.5 SEM gen/period)
(Fig. 2e, f ). Fig. 2 RINGS can assess growth in different bacterial strains
and species. a – c Fluorescence and white light images
of two representative colonies of PAS715 ( E. coli MG1655), PAS716 ( S . Typhimurium LT2), and PAS717
( E. coli Nissle 1917). Scale bars = 0.1 cm. d – f When grown
in log-phase liquid culture, repressilator phase progression
correlated with the estimated generations elapsed as determined
by CFU counts for PAS715 (four biological replicates), PAS716
(three biological replicates), and PAS717 (three biological
replicates). Graphs also show linear regression from combined
means of elapsed phase after IPTG removal. Error bars = 95% CI. Numbers are as follows: PAS715: replicate #1/2/3/4:
0 h:16/76/23/89 2 h:8/14/42/40 4 h:25/15/10/12 6 h:9/11/40/46. PAS716: replicate #1/2/3 – 0 h:145/33/22 2 h:76/43/19
4 h:94/106/18 6 h:32/19/18. PAS717: replicate #1/2/3. 0 h:
116/37/69 3 h: 48/60/96 6 h: 78/41/76 9 h: 48/42 /67. #1–9 h and
#2–6 h data had angular deviation >1.2 and were removed
from downstream analysis. Source data are provided as a Source
Data file Full size image Table 1 Repressilator period lengths calculated by growth in the
mother machine Full size table PAS715 period length remained unperturbed during growth on
extracted mouse cecum contents, used to simulate aspects of the gut environment
(Supplementary Fig. 4a ;
Table 1 ). Similarly, expected growth
variations caused by alternating the presence or absence of the bacteriostatic
antibiotic novobiocin were accurately tracked using RINGS analysis
(Fig. 3 ). Together, these results
indicate that the mechanisms for repressilator 2.0 oscillation are insensitive
to the gene regulation, cell-size, and stress variations under changing species
backgrounds and environmental conditions. This provides confidence both for the
robustness of the RINGS method, and the possibility of extending its use to
other applications and engineerable gut bacterial strains. Fig. 3 RINGS is unaffected by variable bacterial growth. To
test the ability for RINGS analysis to track and integrate
growth under variable conditions, IPTG-synchronized PAS715 was
back-diluted and grown in liquid culture in the presence or
absence of bacteriostatic concentrations of novobiocin. Following 2 h of growth, each culture was washed and split again
to be grown under the presence or absence of novobiocin,
generating four unique combinations of expected growth and
non-growth. The phase of populations sampled at 2 and 4 h were
consistent with the expected growth phenotype. In particular,
the equivalence of the two populations exposed to one period
with and one period without novobiocin, irrespective of order,
demonstrates the ability to measure absolute growth during
periods of variable growth rate. Mean phase ( θ 0 ) from two
independent biological replicates is shown. Numbers of colonies
analyzed per timepoint are as follows: Rep 1/2 – 0 h: 13/20. 2 h
LB: 57/26. 2 h novo: 101/69. 4 h LB-LB: 14/60. 4 h LB-novo:
23/42. 4 h novo-LB: 40/32. 4 h novo-novo: 22/16. Source data are
provided as a Source Data file Full size image RINGS quantifies growth changes within the mouse gut IPTG-synchronized E. coli PAS715
bacteria were delivered by oral gavage to mice that had been treated with a
single dose of streptomycin 24-h prior (Fig. 4a ; replicate: Supplementary Fig. 5a ). Streptomycin-treated mice have been extensively utilized
as a model for E. coli and S . Typhimurium growth in the mouse gut, which is
not a native or permissive host for human-derived E.
coli strains [33] , [34] . We have previously shown that delivery of E. coli to mice that were treated with
single doses of streptomycin affords colonization levels that are initially high
but decrease consistently over the days following [35] , [36] . This likely reflects rapid initial
replication in the niche made available by streptomycin treatment, followed by
progressive recovery of colonization resistance by the native gut and
microbiota [37] . Thus, this model allows us to investigate
the ability for RINGS to detect a range of growth rates within the gut. RINGS
analysis was performed on E. coli PAS715
bacteria isolated from fecal samples (Fig. 4a–d ; replicate: Supplementary Fig. 5a–e ). Repressilator phase remained remarkably
coherent in populations for >20 h after gavage (Fig. 4b ; replicate: Supplementary Fig. 5b, c ). Similar results were found for S . Typhimurium LT2 (PAS716)
(Supplementary Fig. 5g–j ). Fig. 4 The repressilator 2.0 is robust and informative within
the mouse gut. a in vitro
synchronized PAS715 ( E. coli )
bacteria measure growth in mice treated with a single dose of
streptomycin ( n = 3 per
group). b Histograms of
bacterial phase distributions throughout the experiment. Graphs
show normalized counts. 5.75 h timepoint is compared to the
gavage population (black line). Dotted lines represent datasets
with angular deviation >1.2, which were excluded from
downstream analyses. For number of colonies analyzed at each
timepoint, see corresponding data in d . c Graph of
average elapsed phase of the population vs time for each mouse. Graph shows mean with 95% CI. d Cumulative distribution functions of predicted generations
elapsed since gavage. Source data are provided as a Source Data
file Full size image The growth of each species was quantified using the previously
calculated repressilator 2.0 periods (Fig. 2d–f ; Table 1 ), with
physiological constraints for bacterial growth used to assist in the confident
assignment of elapsed growth from RINGS phase data (Supplementary
Fig. 6 ). As expected, RINGS
analysis estimated that growth was most rapid immediately following gavage and
slowed considerably in later timepoints (Fig. 4c , Supplementary Fig. 5d,
i ), with similar average growth predicted for both species
(PAS715: 12.2–15.1 gen and PAS716: 13.0–15.1 gen at 20.5 h post gavage). 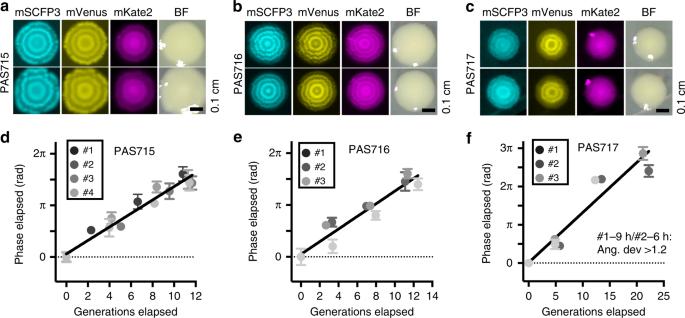Fig. 2 RINGS can assess growth in different bacterial strains
and species.a–cFluorescence and white light images
of two representative colonies of PAS715 (E. coliMG1655), PAS716 (S. Typhimurium LT2), and PAS717
(E. coliNissle 1917).
Scale bars = 0.1 cm.d–fWhen grown
in log-phase liquid culture, repressilator phase progression
correlated with the estimated generations elapsed as determined
by CFU counts for PAS715 (four biological replicates), PAS716
(three biological replicates), and PAS717 (three biological
replicates). Graphs also show linear regression from combined
means of elapsed phase after IPTG removal. Error bars = 95% CI.
Numbers are as follows: PAS715: replicate #1/2/3/4:
0 h:16/76/23/89 2 h:8/14/42/40 4 h:25/15/10/12 6 h:9/11/40/46.
PAS716: replicate #1/2/3 – 0 h:145/33/22 2 h:76/43/19
4 h:94/106/18 6 h:32/19/18. PAS717: replicate #1/2/3. 0 h:
116/37/69 3 h: 48/60/96 6 h: 78/41/76 9 h: 48/42 /67. #1–9 h and
#2–6 h data had angular deviation >1.2 and were removed
from downstream analysis. Source data are provided as a Source
Data file These
dynamics were further confirmed by Peak-to-Trough Ratio (PTR) analysis, which
estimates the average instantaneous growth rate of a population from metagenomic
sequencing data (6 h: 1.72 ± 0.08, n = 4;
>16 h: 1.44 ± 0.08, n = 9;
Supplementary Table 2 ) [15] . Together these data demonstrate the
ability for RINGS to detect changing growth within the mouse gut. In vivo repressilator 2.0 control and stability To allow in vivo control of the repressilator 2.0 circuit and
re-gain synchronicity of the bacterial populations growing within the mouse gut,
mice carrying asynchronous PAS715 bacteria were provided IPTG or aTc in their
drinking water (Fig. 5a ). RINGS analysis
on fecal samples in pre- and post-synchronized mice clearly demonstrated the
ability to synchronize the repressilator within the mouse gut (Fig. 5b ). Fig. 5 The repressilator 2.0 can be controlled in situ within
the mouse gut. a Mice
( n = 2 per group)
carrying asynchronous PAS715 were provided IPTG or aTc in
drinking water to synchronize the repressilator. b RINGS analysis demonstrated the
progression from pre- (top) to post-synchronization (bottom). Graph shows histograms of normalized phase count distributions. Numbers are as follows: IPTG1/2—pre: 133/97. Post: 172/206. aTc1/2—pre:149/114. post: 213/193. c . Repressilator in situ synchronization allows
RINGS analysis following initial colonization, with bacteria
plated on selective plates to assay for repressilator and sponge
plasmid retention, or RINGS analysis to follow repressilator
phase. After 15 days, provision of streptomycin in drinking
water overnight selected remaining PAS715 bacteria to allow
isolation and imaging of colonies that had been continually
present in the gut. d Plasmid
retention (colored samples, left axis) and bacterial abundance
(black samples, right axis) data from plating on differentially
selective plates. Graph shows individual values and mean line. Numbers are as follows: rep1/2 – 20 h: 772/443. 42 h: 1041/905. 68 h: 1967/1742.102 h: 585/841. e Fluorescence and white light images of two
representative colonies of PAS715 isolated 16 days post gavage. Scale bars = 0.1 cm. f RINGS
analysis of phase progression 42 h (0 h post sync) -102h (60 h
post sync) after gavage. Graphs show histograms of normalized
bacterial phase count distributions. For number of colonies
analyzed at each timepoint, see corresponding data in g . g Cumulative distribution functions of predicted
generations elapsed since gavage. Source data are provided as a
Source Data file Full size image The repressilator circuit was stable over extended periods of
growth in the gut. To test plasmid retention, E.
coli PAS715 bacteria were provided to mice previously treated
with a single dose of streptomycin. Plating of fecal samples was then used to
identify plasmid loss events within the bacteria (Fig. 5c ). Retention of both the repressilator 2.0 plasmids
remained high for >100 h in the mouse gut (80–88% retention at 102 h
post gavage), indicating that the repressilator circuit can remain active over
these time frames (Fig. 5d ). Furthermore, functional PAS715 colonies could still be isolated 16 days after
first entering the gut (Fig. 5e ),
demonstrating the potential for this synthetic circuit to maintain longer-term
oscillatory gene expression in a competitive environment. Long-term in vivo growth determination using RINGS Repressilator 2.0 circuit stability and in situ synchronization
capacity allows for long-term growth determination. To measure growth after
initial establishment in the gut, during plasmid retention testing PAS715
bacteria were synchronized in situ with IPTG (Fig. 5c ). Based on our findings that bacterial growth slowed over
the initial 24-h period (Fig. 4a–d ,
Supplementary Fig. 5a–e ) RINGS
analysis was performed beginning the day after IPTG removal on fecal samples
taken ~daily, with well under a single period of growth expected between each
timepoint (Fig. 5f ). Repressilator phase
remained coherent (Fig. 5f ) predicting
6–12 generations (IPTG 3, 90% CI) and 5–9 generations (IPTG 4, 90% CI) of growth
over the 60-h period beginning ~2 days after gavage (Fig. 5g ). RINGS detects disease and niche-specific growth variations Different growth behavior was determined in the inflamed gut and
between regions of the gut. Repressilator-bearing PAS715 bacteria were
introduced into dextran sulfate sodium (DSS) -treated animals as a model for
inflammation, which promotes increased growth of Enterobacteriaciae [38] , [39] (Fig. 6a ). Bacterial populations retrieved from the feces of
DSS-treated mice 15 h after delivery showed greater phase heterogeneity than
those from streptomycin-treated control mice (Fig. 6b ), as demonstrated by comparison of the angular deviation,
the circular statistical analogue to standard deviation, of each population
(strep control: 0.9 ± 0.0 SEM, n = 4;
DSS-treated: 1.1 ± 0.1 SEM, n = 4)
(Fig. 6c ). These results were
consistent with previous experiments that showed signs of decoherence of PAS715
populations <20 h in the inflamed gut (Supplementary Fig. 7a, b ). DSS (4%) did not affect the
repressilator during in vitro growth (Supplementary Fig. 7c ) and repressilator 2.0 period length was not
affected by growth on cecum contents extracted from either untreated or DSS-fed
mice (Table 1 ). Together these results
suggest that the DSS-inflamed gut provides a more heterogeneous growth
environment than the streptomycin-treated gut. Fig. 6 RINGS identifies increased growth variability in the
inflamed gut and between gut niches. a RINGS was used to compare PAS715 growth
between the dextran sulfate sodium (DSS) inflamed, or
streptomycin treated, mouse gut. b Histograms of normalized bacterial phase
counts in gavage (black and grey) and fecal samples extracted
15 h post gavage in streptomycin (green) and DSS (red) treated
mice c Bacteria extracted from
feces of DSS-treated mice (red) showed elevated RINGS
variability compared to gavage (black) and streptomycin (green)
treated mice. Graphs show angular deviation of each datapoint
and mean. Arrows identify mice dissected and analyzed in e . d Quantification of LCN-2 in feces 15 h post
gavage demonstrates elevated inflammation in DSS-treated mice. e Bacteria plated from the
dissected mouse gut of streptomycin control (top; n = 1) and DSS-treated (bottom; n = 1) mice. Graphs show
histograms of normalized bacterial phase counts from populations
dissected from regions of the gut (various colors) and feces
(brown) compared to the original gavage (black). Source data are
provided as a Source Data file Full size image Interestingly, despite all DSS-treated mice showing equivalent
severity of inflammation, as measured by lipocalin 2 (LCN-2) levels
(Fig. 6d ), PAS715 remained
relatively synchronous in one of the DSS-treated mice, with an angular deviation
of the fecal population similar to that seen in streptomycin-treated mice
(Fig. 4c , arrow). To further analyze
bacterial growth within this mouse, we dissected the lower gastrointestinal
tract and separately plated bacteria extracted from distinct regions of the gut:
ileum, cecum, proximal colon lumen, proximal colon mucus, distal colon lumen,
distal colon mucus, and feces (Fig. 6e ). Dissection analysis of a streptomycin control mouse showed similar RINGS phase
distributions for all regions measured (Fig. 6e , top). By comparison, populations extracted from the
DSS-treated mouse showed similar RINGS phase distributions in all regions except
the ileum, which was distinctly phase shifted (Fig. 6e , bottom). Thus, even when not reflected in feces, greater
PAS715 growth heterogeneity was evident in the DSS-treated compared to
streptomycin-treated gut. The difference in growth elapsed between bacteria in
the ileum and the remainder of the DSS-treated gut is a likely cause for the
increased growth variability we detect in fecal samples from other DSS-treated
mice. Here we describe the activity of a synthetic gene oscillator, the
repressilator 2.0, in the complex environs of the mammalian gut. We develop an image
processing and analysis pipeline, RINGS, to follow repressilator activity on a
single-cell level and thereby also understand growth dynamics at various stages of
the colonization process. We demonstrate robust repressilator 2.0 functionality,
control and circuit stability within the mouse gut over the course of several days. Using this method we detect increased growth variability under inflammatory
conditions and between spatial niches within the gut The repressilator 2.0 is ideally suited to periodic expression control
within engineered bacteria for use in complex settings. The circuit’s independence
from external signals allows for circuit function in a variety of environments,
which is of particular utility in the gut where relative abundance of strains can
vary widely on spatial and temporal scales, and between individuals. To this end,
the ability to re-synchronize the repressilator 2.0 in situ within the gut, and its
stability over extended periods of growth without antibiotic selection are
particularly exciting. The RINGS method informs us of the integrated growth experience of a
bacterium and its forebears. The repressilator 2.0’s periodicity allows for extend
growth measurement in comparison to other comparable techniques, recent examples of
which include a synthetic particle which allows mark-and-recapture analysis over ~14
generations [30] , and fluorescent protein dilution which is
capable of estimating up to ~10 divisions of single-cell
growth [21] . Our analyses estimated E. coli MG1655 division times progressively increasing from ~35 min,
when colonizing the recently streptomycin-treated gut, to ~20 h when more removed
from the perturbation of the single dose of streptomycin and thus reflecting more
physiological growth conditions. By comparison, a recent study used the accumulation
of mutations in the E. coli genome to estimate a
division time in humans of 15 h [40] . Together, our results suggest that the aggregate bacterial experience
is relatively consistent under most scenarios tested, with spatial dissection
suggesting that the majority of growth in these mouse colonization models is
occurring ‘upstream’ in the small intestine and/or cecum. We see that in most cases
fecal sampling accurately reflected the overall growth profile of the mouse colon,
including bacteria in the lumen and mucus layers, and within the cecum. The absence
of colonies in fecal samples reflecting the differential growth observed in the
ileum of the dissected DSS-treated mouse suggests that, in this case at least, the
bacteria from the ileum either were not represented in feces or represent a small
enough percentage of the population so as to remain below detection in our final
analyses from this mouse. Overall, we determine that single-cell measurements are particularly
important in disease conditions, such as inflammation, when variability of growth
between niches is accentuated. In these cases methods that can only measure a
population-wide average would not adequately represent the population’s diversity. The ability to increase the sampling frequency used would also allow this method to
measure the emergence of subpopulations of differentially growing bacteria in finer
detail. In sum, analysis of the repressilator at single-cell level can report
on complex bacterial growth behaviors over time, and in particular, during disease
conditions within the mammalian gut. In doing so, this work demonstrates the
potential for one of the circuits that first stimulated the field of synthetic
biology to revolutionize how we control gene expression within the gut. 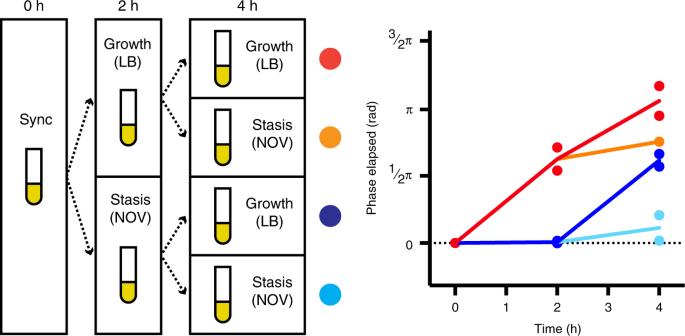Fig. 3 RINGS is unaffected by variable bacterial growth. To
test the ability for RINGS analysis to track and integrate
growth under variable conditions, IPTG-synchronized PAS715 was
back-diluted and grown in liquid culture in the presence or
absence of bacteriostatic concentrations of novobiocin.
Following 2 h of growth, each culture was washed and split again
to be grown under the presence or absence of novobiocin,
generating four unique combinations of expected growth and
non-growth. The phase of populations sampled at 2 and 4 h were
consistent with the expected growth phenotype. In particular,
the equivalence of the two populations exposed to one period
with and one period without novobiocin, irrespective of order,
demonstrates the ability to measure absolute growth during
periods of variable growth rate. Mean phase (θ0) from two
independent biological replicates is shown. Numbers of colonies
analyzed per timepoint are as follows: Rep 1/2 – 0 h: 13/20. 2 h
LB: 57/26. 2 h novo: 101/69. 4 h LB-LB: 14/60. 4 h LB-novo:
23/42. 4 h novo-LB: 40/32. 4 h novo-novo: 22/16. Source data are
provided as a Source Data file Strains, plasmids, and bacterial culturing Details of strains (Supplementary Table 1 ) and plasmids (Supplementary Table 3 ) used in this study are provided. The repressilator 2.0 plasmid variant with three fluorescent
reporters (pLPT234) was constructed by isothermal
assembly [41] by combining PCR products from previously
published degradation-tag free repressor genes—Tn10 transposon derived tetR , bacteriophage λ derived cI and E. coli lactose operon derived lacI (pLPT119)—and
triple fluorescent reporters—P R -mKate2 (including the
first 11 amino acids of mCherry for improved translation efficiency as
previously published [5] ), P LtetO1 –mVenus,
P LlacO1 –mSCFP3 (pLPT107) [5] . Previously published
sponge plasmid variants [5] were used as available from Addgene
plasmid repository (see Data Availability Statement). Plasmids were isolated by
miniprep (Qiagen) and were routinely transferred to new strains as a mixture by
electroporation. To avoid interruption of the repressilator and ensure clear ring
development within colonies, lacI and motA genes were knocked out of E. coli strains used before repressilator plasmids
were transferred. For both genes, FRT-flanked gene disruption constructs were
transferred by P1 vir transduction [42] from the relevant Keio collection
strains [43] . Kanamycin resistance genes were then
removed by electroporation and subsequent curing at 43 °C of
pCP20 [44] . Similarly, streptomycin resistance based on
a rpsL lys42arg mutation was transferred by
P1 vir from a previously generated E. coli MG1655
strain [35] . Resistance to streptomycin was evolved in S . Typhimurium LT2 by serial passage in
liquid culture with increasing concentrations of streptomycin sulfate (Sigma)
(50,100, 200, 300 μg/mL). For PAS718, mKate2 (including the first 11 amino acids
of mCherry for improved translation efficiency as previously
published [5] ) driven under the
P RNA1 constitutive promoter was inserted into the
genome using a Tn7 transposon [45] , and acted as a constitutive fluorescent
marker for cell segmentation in mother-machine experiments. Bacteria were routinely cultured in Luria broth (LB) supplemented
with 300 μg/mL streptomycin (Sigma), 100μg/mL carbenicillin or ampicillin
(Sigma) and 50μg/mL kanamycin (Sigma). For plating, bacteria were grown on
selective LB agar plates supplemented with 100μg/mL carbenicillin (Sigma) and
50μg/mL kanamycin (Sigma). The plasmid retention test compared growth on
streptomycin (all PAS715 derivatives) to streptomycin+carbenicillin (retention
of repressilator plasmid), streptomycin+kanamycin (retention of sponge plasmid),
and streptomycin+carbenicillin+kanamycin (retention of both plasmids) at drug
concentrations as above. To synchronize the phase of the repressilator across the
population, bacteria were grown overnight in the presence of 1 mM Isopropyl
β-D-1-thiogalactopyranoside (IPTG) (Sigma) or 100 nm anhydrotetracycline (aTc)
(Sigma). Bacteria were back-diluted in fresh inducer-supplemented media by at
least 1:20 to allow resumption of active growth in the presence of inducer,
before being washed and utilized for downstream experiments. Colony imaging Fluorescent and white light images of colonies were imaged using a
custom-software controlled Canon T3i digital single lens reflex (DSLR) camera
with a Canon EF-S 60 mm USM lens, combined with LEDs and filters for excitation
and a Starlight express emission filter wheel (CFP: 440–460 nm LED with 436/20
EX and 480/40 EM filters; YFP: 490–515 nm LED with 500/20 EX and 530/20 EM
filter; RFP: 588–592 LED with 572/35 EX and 645/75 EM filter; white: 3500–4500 K
LED) [46] . Images were taken at an aperture of f/2.8
and ISO200. Exposure times were typically between 0.05 and 2 s as experimentally
determined to maximize dynamic range. Generative model development for RINGS phase profiling We extract the relative phase offset of each colony by fitting a
generative model to the pattern of oscillations. This approach has the benefit
of making use of all the information captured in the multi-channel images. We
explored a family of generative models, based on the simple form: 
    I = Asin( f( r )) + B
 (1) where A and B are the amplitude and offset of a sinusoidal
oscillator, and the function, f ( r ), represents the radial phase profile of the
colony. The form of f ( r ) is derived below using a simple model for the growth of the
colonies. The phase profile, f ( r ), is related to the profile of generation number, g ( r ),
as follows: 
    f( r ) = 2π/Tg( r) + θ _0
 (2) where T is the period of the
oscillator in generations (≈ 15.5) and θ 0 is the instantaneous phase of the
oscillator at the time of plating. Thus, we derive the profile of generation
number with respect to radius. We assume that growth is initially exponential,
and then becomes restricted to an annulus with thickness D (≈30 μm at the edge of the colony [40] ). Assuming uniform packing of bacteria in the colony (for both phases
of growth), the generation number profile during exponential growth can be
derived simply: 
    g( r ) = log( π/A_br^2)/log( 2 )
 (3) where A b is
the area of a single bacterium Here we model the growth of the colony with each successive
generation. With each generation the radius of the colony increases as
follows: 
    Δr/Δg = r( √(1 + 2D/r - ( D/r)^2 - 1))
 (4) Integrating this over the colony, we obtain the following
expression for the generation number profile: 
    [ g( r ) = 1/4D[ 2r( 1 + a( r )) + 2Dlog( 2r - D) + 3Dlog( D + r( 1 + a( r ))). ;                                . - Dlog(  - D + r( 3 + a( r )))] + g_0 ]
 (5) g o is the
generation number at the transition between the exponential and annular
growth. Combining the two growth models yields a continuous growth curve
(Supplementary Fig. 8 ). We set the
transition between the exponential and annular growth at r = D , with D = 30 μm. Notice that beyond r ≈ 100 μm the phase profile is approximately
linear, and can be described by: 
    f( r ) = ( 2π/DT)r + θ _0
 (6) We checked this result by measuring the slope for the phase profile
directly from images of colonies. The distance between two peaks in any given
colony is ~490 μm, yielding a phase profile with slope 0.0128 rad/μm. Using an approximate value of 15.5 generations per cycle,
Eq. 6 predicts an annulus size, D ≈ 32 μm, consistent with the ≈30 μm
growth annulus reported in previous studies [47] . Thus, we model the phase profile of a bacterial colony using
Eq. 1 with a linear phase profile,
described by Eq. 6 . Image preprocessing Centered colonies were cropped from whole-plate images using
FIJI [48] . Color images from single fluorescent
exposures in CFP and YFP channels were imported, and the relevant spectral
component image utilized for downstream processing (CFP—blue channel, YFP—Green
channel). Colonies were identified by autothresholding (Yen method) of binarized
CFP images. Separate YFP and CFP images were cropped and exported, centered on
the YFP center of mass of each identified colony. Prior to final analyses,
colony images from plates containing >130 bacterial colonies were
excluded based on overcrowding leading to limited colony growth. Remaining
colonies were visually inspected, and any doublet or severely malformed colonies
were removed from the datasets to avoid spurious fitting. Colony removal was
performed blinded to θ 0 fit values. Where presented, average
projections were taken through YFP images from all colonies identified in a
given population. RINGS generative model fitting Preprocessed colony images were normalized for global changes in
intensity, before fitting the model described above. We observed that in each
colony, the expression of YFP and CFP decayed dramatically with increasing
radius. To compensate for this decay, the images were masked at radius of r max = 1.3 mm
( r max = 1.1 mm for S . Typhimurium colonies, which were
commonly smaller) and the radial intensity profile was fit to a second order
polynomial. This smooth polynomial decay, chosen as an even order with negative
coefficient to ensure this process did not remove the oscillatory pattern, was
then used to normalize the raw image in a pixel-wise fashion (Supplementary
Fig. 9 ). We also explored
normalization with a fourth order polynomial, but this was deemed less
appropriate. For multi-channel images, the polynomial functions shared
parameters for the center of the colony, but each channel was fit to its own
decay profile. To fit the oscillatory pattern of a single colony, we use
Eq. 1 with a linear phase profile. However, we allow for both the slope and offset of the phase profile to be fit
(Eq. 6 ), as well as the amplitude
and offset of the intensity (Eq. 1 ). The
slope for the phase profile is initialized to an expected value that varies
based on strain, and the phase offset is initialized to zero. We tested
optionally masking the central region of the colony, to account for the early
exponential growth phase, which we do not attempt to model, however, found no
benefit to fit based on this. Fitting is done in Matlab using the
Levenberg-Marquardt (LM) algorithm (Supplementary Fig. 9 ). The fitting routine returns the center position of the colony, the
amplitude and offset of the oscillations, as well as the slope and offset of the
phase profile. The phase offset is the property of interest. However, fitting
the radial expression profile is challenging due to numerous local minima in the
error surface. Thus, we filter out colonies for which the slope of the phase
profile, or the inferred center position of the colony is outside of an accepted
range. We also explored the use of robust error functions, to minimize the
effect of asymmetric bright patches of expression in the colony, as well as
weighted nonlinear regression to compensate for the increasing number of pixels
at increasing radius. However, neither of these approaches greatly improved upon
the LM algorithm, which we used by default. We also explored fitting phase
profiles with higher order polynomials; however, we found this to be very
unstable. Fitting was improved by simultaneous regression in multi-channel
images. In this case, the phase offset of the two channels was fixed to a
constant value. We found that YFP oscillations lead CFP by a strain-specific
value. Thus, we regressed the slope and offset of the phase profile using both
channels, with a fixed phase difference between the two channels, as calculated
for each strain. See Eq. 7 and 8 . I_YFP = A_YFPsin( kr + θ _0 + strain offset) + B_YFP
 (7) 
    I_CFP = A_CFPsin( kr + θ _0) + B_CFP
 (8) RINGS method parameter testing We tested the performance of this method by applying it to in vitro
timecourse data where colony counts could be used to provide a known average
generation shift between each timepoint. Parameter sweeps were performed on key
parameters expected to vary between strains, particularly the size of colony
mask (‘rMax’), the distance between each ring and therefore expected slope of
the phase profile (‘expectedSlope’), the variation in slope between colonies
(‘slopeTol’), and the offset between CFP and YFP rings (‘colorPhaseShift’). The
method was found to be largely insensitive to specific parameter values with
strain-specific optimal values likely caused by differences in oscillator and
spatial colony growth characteristics. Optimal parameters for each strain in the
study were determined to be as follows: (LPT320: ‘rMax’:1.3, ‘expectedSlope’:
0.39, ‘slopeTol’: 0.3, ‘colorPhaseShift’: 1.5. PAS715: ‘rMax’:1.3,
‘expectedSlope’: 0.34, ‘slopeTol’: 0.4, ‘colorPhaseShift’: 0.9. PAS716: ‘rMax’:
1.1, ‘expectedSlope’: 0.43, ‘slopeTol’: 0.4, ‘colorPhaseShift’: 1.0. PAS717:
‘rMax’:1.3, ‘expectedSlope’: 0.41, ‘slopeTol’: 0.3, ‘colorPhaseShift’:
0.83.). Statistical analyses Statistical analyses were performed in MATLAB versions R2017a-2018a
(Mathworks) or Prism v6-7 (Graphpad). Circular statistical tests, specifically
circular mean and angular deviation, were performed using the CircStat for
Matlab toolbox v2012a [49] . Briefly, to calculate circular mean, θ 0 values are transformed to a resultant
mean vector (Eq. 9 ). 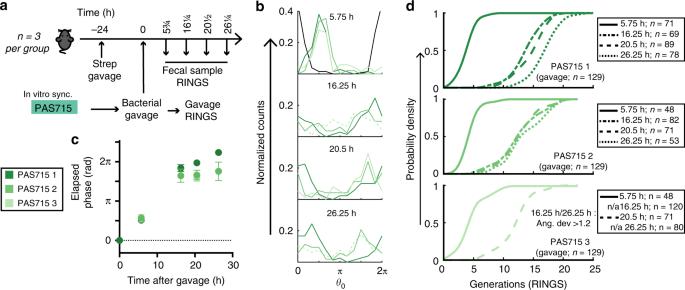Fig. 4 The repressilator 2.0 is robust and informative within
the mouse gut.ain vitro
synchronized PAS715 (E. coli)
bacteria measure growth in mice treated with a single dose of
streptomycin (n= 3 per
group).bHistograms of
bacterial phase distributions throughout the experiment. Graphs
show normalized counts. 5.75 h timepoint is compared to the
gavage population (black line). Dotted lines represent datasets
with angular deviation >1.2, which were excluded from
downstream analyses. For number of colonies analyzed at each
timepoint, see corresponding data ind.cGraph of
average elapsed phase of the population vs time for each mouse.
Graph shows mean with 95% CI.dCumulative distribution functions of predicted generations
elapsed since gavage. Source data are provided as a Source Data
file 𝐫 = sum( exp( iθ _0))
 (9) The circular mean, α , is then
calculated from this vector (Eq. 10 ). α = angle( 𝐫)
 (10) Angular deviation, s , is a
circular statistical analogue of linear standard deviation. It is derived from
the length of the resultant mean vector (Eqs. 11 and 12 ). Angular
deviation values are bounded, lying between 0 and √2. Conceptually, this occurs
because values equally spread around the unit circle are maximally
spread. R = 𝐫
 (11) 
    s = √(2( 1 - R))
 (12) Elapsed phase measurements Downstream processing of phase measurements was predominantly
undertaken using custom scripts in Matlab versions 2016a–2018a. In order to
estimate the total phase elapsed during an experiment, we made the assumption
that repressilator phases across the population fell within ±π of the circular
mean (i.e., we assumed that all colonies lie within ~15 generations elapsed of
each other). We deemed this appropriate where the population remained relatively
coherent around the circular mean—which we defined as having an angular
deviation <1.2. Empirically, datasets with angular distribution
>1.2 were routinely decoherent, were not accurately described by the
circular mean (e.g., in cases of a bifurcated population), or contained
considerable fractions of the population in regions neighboring the mean ± π
divide, which reduced our confidence of accurately classifying these cells as
being slower or faster growing (Supplementary Fig. 10 ). While in many cases valuable insight may still be gained
by further analysis on a case-by-case basis, particularly when taken in the
context of other datapoints or experimental replicates, we conservatively
elected to restrict our interpretations of such datasets to the raw θ 0 data, which are
unaffected by this. For elapsed phase calculations, individual phase values ( θ 0 ) were normalized to the
circular mean of the initial synchronized repressilator 2.0 population for that
experiment, α sync . Elapsed phase was then calculated by addition/subtraction of multiples of 2π
based upon the circular mean of a timepoint. When α n > α n-1 i.e., when growth had occurred but not, on average, passed the 2π/0 point, the
adjustment factor remained unchanged. However, when α n < α n-1 ,
i.e., growth on average passed the 2π/0 divide within the elapsed timepoint, an
adjustment factor of 2π was made to each subsequent timepoint. When this method
was applied to in vivo datasets, where sampling variability combined with slow
growth rates could lead to spurious negative shifts, we further assumed that
average growth rates would not exceed 2.5 generation per hour when interpreting
if a population had grown through a full period. Individual θ 0 values were then adjusted
by addition of the calculated multiples of 2π. For adjustments, where \({\bar{\alpha}}\) < π, colonies with θ 0 = α − π to 0 were assumed to be one phase revolution (i.e., 2π
radians) behind of those of 0 to α + π. Where α > π, colonies with θ 0 = 0 to α − π were assumed
to be one phase revolution ahead of values α − π to 0. Subsequent
calculations treated the adjusted θ 0 values as linear datasets. To calculate growth on a single-cell level we treated each colony
separately, determining the distribution of probability for the generations of
growth since the reference timepoint ( t sync ) on a single-cell basis. Because
adjusted θ 0 values had
already been normalized to α sync = 0 and adjusted for multiple periods of growth
where necessary, the mean estimated growth, μ , for each individual colony in the population, i , is described by: 
    μ _i = θ _0( adjusted) i/2π×period_strain
 (13) where period strain is the calculated mean
periodicity of the relevant strain in generations/period. The distribution of probable growth can then be determined by a
combination of the phase distribution of the population at
t sync and the uncertainty in our periodicity
measurements. Initial synchronized repressilator 2.0 populations
(t sync ) were assumed to be normally distributed,
which was appropriate based on visual inspection of Q–Q plots. Thus, the growth
probability of each colony, i, is described by a normal distribution with
error,σ: 
    σ _i = μ _i√(( period error/period_strain)^2 + ( σ _tsync/θ _0( adjusted)i)^2)
 (14) An empirical probability density function and cumulative
distribution function was then calculated as the sum of all individual
distributions. Interpretations of growth data are informed by physiological
limits. For example, we can assume that growth will not exceed known growth
rates for a given species, and the repressilator can only progress in one
direction based on growth. Of the possible outcomes, we report the most
consistent growth trajectory across timepoints. An example of how these
constraints are applied to a dataset is provided (Supplementary
Fig. 6 ). Histograms For histograms, θ 0 data were separated into π/6-width
bins centered on 0 and multiples of π/6. Counts were normalized by the total
number of fit colonies in each dataset. Datapoints were plotted at each bin
center. For linear histograms, 0 and 2π are plotted as the same value. In vivo bacterial growth testing The Harvard Medical School Animal Care and Use Committee approved
all animal study protocols and all experiments complied with relevant ethical
regulations. Female C57Bl/6 (Jackson Laboratory) mice of 8–14 weeks, (including
>2 weeks acclimatization to the HMS mouse facility), were used in groups
of 2–3 per experiment. Mice were routinely randomized between treatment groups
in advance of experiments, where relevant. Mice were fed on a lactose-free chow
(Envigo Teklad Global 18% Protein Rodent Diet) for at least 1 week prior to
provision of repressilator bacteria to avoid any interruption of the
repressilator by lactose. Streptomycin-treated mice were administered 5 mg
USP-grade streptomycin sulfate (Gold Biotechnology) in 100 μL sterile PBS by
oral gavage, or where specifically stated 0.5 g/L in drinking water supplemented
with 5% sucrose overnight. PAS715 E. coli MG1655 bacteria or PAS716 S . Typhimurium LT2
bacteria were prepared for administration by pelleting from culture, washing and
dilution in sterile PBS before provision to mice as a 100μL oral gavage. In situ synchronization was achieved by provision of USP-grade
10 mM IPTG (Sigma) or 0.1 mg/mL aTc (Sigma) in drinking water supplemented with
5% sucrose overnight. Fresh fecal samples were collected by temporarily removing mice to
small containers until at least 2–3 fecal pellets were produced. Fecal pellets
were homogenized in PBS at 50 or 100 mg/mL in sterile PBS by vortexing for
~5 min in 1.5 mL Eppendorf tubes. To remove large debris, homogenized feces was
then centrifuged either by briefly pulsing (~1 sec) on a benchtop minifuge
(where CFU counts were not critical), or by centrifugation at 4 × g for 20 min (where CFU counts were critical). The
supernatant was then serially diluted and cultured on selective agar
plates. For inflammation experiments, mice were fed Dextran Sulfate Sodium
(Colitis Grade, M.W. = 36,000–50,000, MP Biomedicals, LLC) in drinking water
supplemented with 5% sucrose for 3 days prior to bacterial administration. DSS
water was exchanged every second day, and mice remained exposed throughout the
course of the experiment. LCN-2 biomarker levels [50] were quantified as
previously [36] using a Mouse lipocalin-2/NGAL DuoSet ELISA
kit (R&D Systems). Fecal pellets were vortexed at 100 mg/mL in PBS+0.1%
Tween20 for 20 min, then pelleted at 12,000 × g for 10 min at 4 °C. ELISA results were obtained on a BioTek
Synergy H1 plate reader. Four hundred fifty nanometer absorbance corrected
values were interpolated from a sigmoidal four parameter logistic standard curve
using Prism 7 for Mac OSX software (GraphPad). Peak-to-trough ratio analysis Peak-to-trough ratios were computed from metagenomic sequencing of
mouse fecal samples as previously described [15] . Genomic DNA was
extracted from flash-frozen fecal samples using a Qiagen DNEasy Blood &
Tissue Kit. Genomic DNA from each sample was prepared for sequencing using a
Kapa HyperPlus Kit and sequenced using an Illumina NextSeq at the Bauer Core
Facility at Harvard University. Sequencing reads were trimmed for quality using
Trimmomatic 0.36 [51] and each sample was aligned to the genome of
interest using BWA mem 0.7.8 [52] . Sequencing coverage was obtained using
bedtools 2.27.1 [53] . To calculate peak-to-trough ratio, mean
coverage was computed for 10 kb bins across the genome and a segmented linear
model was fit to the coverage using the R package
segmented [54] . Growth in the mother machine We performed time-lapse single-cell measurements to monitor and
compare the dynamics of repressilator circuits in rich defined medium (EZ Rich
Defined Medium; Teknova) and in cecum contents. Cecum contents were derived from
fresh or frozen mouse cecum, diluted in PBS. 2–4 FVB (Charles River) or C57/Bl6
(Jackson) mice were sacrificed, their cecum dissected, and the cecum contents
were extracted by scraping and washing off the tissue with PBS. When frozen,
cecum contents were placed at −80 °C. The contents were then thawed, if
necessary, and diluted in PBS, spun briefly in a benchtop centrifuge
(13,000 × g ) to remove large particulate
matter and the supernatant removed and saved. Cecum matter was then washed a
second time, centrifuged, and the supernatant pooled with the first wash. Pooled
supernatant was centrifuged a second time, then passed sequentially through a
20 μm syringe filter (Millex-AP glass fiber 25 mm syringe filter) and then a
5 μm syringe filter (Pall Acrodisc 32 mm syringe filter with 5 μm
Supor ® membrane). 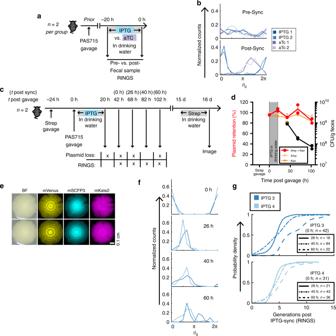Fig. 5 The repressilator 2.0 can be controlled in situ within
the mouse gut.aMice
(n= 2 per group)
carrying asynchronous PAS715 were provided IPTG or aTc in
drinking water to synchronize the repressilator.bRINGS analysis demonstrated the
progression from pre- (top) to post-synchronization (bottom).
Graph shows histograms of normalized phase count distributions.
Numbers are as follows: IPTG1/2—pre: 133/97. Post: 172/206.
aTc1/2—pre:149/114. post: 213/193.c. Repressilator in situ synchronization allows
RINGS analysis following initial colonization, with bacteria
plated on selective plates to assay for repressilator and sponge
plasmid retention, or RINGS analysis to follow repressilator
phase. After 15 days, provision of streptomycin in drinking
water overnight selected remaining PAS715 bacteria to allow
isolation and imaging of colonies that had been continually
present in the gut.dPlasmid
retention (colored samples, left axis) and bacterial abundance
(black samples, right axis) data from plating on differentially
selective plates. Graph shows individual values and mean line.
Numbers are as follows: rep1/2 – 20 h: 772/443. 42 h: 1041/905.
68 h: 1967/1742.102 h: 585/841.eFluorescence and white light images of two
representative colonies of PAS715 isolated 16 days post gavage.
Scale bars = 0.1 cm.fRINGS
analysis of phase progression 42 h (0 h post sync) -102h (60 h
post sync) after gavage. Graphs show histograms of normalized
bacterial phase count distributions. For number of colonies
analyzed at each timepoint, see corresponding data ing.gCumulative distribution functions of predicted
generations elapsed since gavage. Source data are provided as a
Source Data file 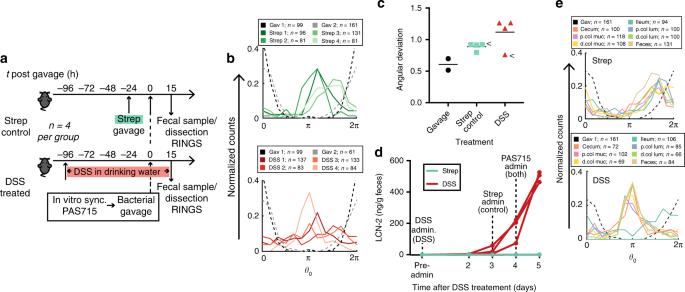Fig. 6 RINGS identifies increased growth variability in the
inflamed gut and between gut niches.aRINGS was used to compare PAS715 growth
between the dextran sulfate sodium (DSS) inflamed, or
streptomycin treated, mouse gut.bHistograms of normalized bacterial phase
counts in gavage (black and grey) and fecal samples extracted
15 h post gavage in streptomycin (green) and DSS (red) treated
micecBacteria extracted from
feces of DSS-treated mice (red) showed elevated RINGS
variability compared to gavage (black) and streptomycin (green)
treated mice. Graphs show angular deviation of each datapoint
and mean. Arrows identify mice dissected and analyzed ine.dQuantification of LCN-2 in feces 15 h post
gavage demonstrates elevated inflammation in DSS-treated mice.eBacteria plated from the
dissected mouse gut of streptomycin control (top;n= 1) and DSS-treated (bottom;n= 1) mice. Graphs show
histograms of normalized bacterial phase counts from populations
dissected from regions of the gut (various colors) and feces
(brown) compared to the original gavage (black). Source data are
provided as a Source Data file The filtered fluid was then
used as an input for the mother machine. The filtered fluid from the cecum contents was loaded in 10 mL
syringes and pumped through mother-machine devices [32] using a Higher Pressure
Programmable Syringe Pump (NE1000). To flow the cecum through the device, we
used a mother-machine design where the dimensions of the flow channel has been
optimized for flowing dense cultures and maintaining low pressure to allow low
fluid flow-rates (Bakshi, S., Leoncini, E., Baker, C., Cañas-Duarte, S.J.,
Okumus, B. and Paulsson, J., personal communication). Device fabrication used a
wafer prepared using standard UV photolithography, with quartz-chrome photomasks
(Toppan Inc) in a clean-room environment. Devices consisted of three independent
layers: a Su8 ‘base’ coat, a featureless uniform layer of completely cured Su8;
cell channels (25 μm long, 1.5 μm wide, and 1.3 μm height) placed in the
orthogonal direction to the flow channels; and medium flow channels, of 150 μm
width and 45 μm height. The devices were constructed from the wafer using soft lithographic
techniques in clean-room (Harvard Medical School Microfabrication Core). Dimethyl siloxane monomer (Sylgard 184) was mixed with curing agent (10:1
ratio), defoamed, poured onto the silicon wafer, degassed (1 h) and cured at
65°C (1 h). Individual chips were cut and the inlets and outlets punched with a
biopsy puncher. On the day of experiments, bonding to KOH-cleaned cover slips
was done using oxygen plasma treatment (30 sec at 50 W and
O 2 pressure at 170 mTorr). Chips were incubated at
95 °C, >30 min to reinforce bonding before being cooled to
room-temperature. Cell channels were loaded with E. coli containing the repressilator
circuit. In some experiments E. coli PAS718,
constitutively expressing mKate2, was used, with the mKate2 acting as a marker
to segment single cells and to extract intensities and cell-growth estimates
more effectively. We used a slow flow-settings (5 μL/min) to ensure we
could observe the dynamics of the cells for prolonged periods (>10 h)
with the small volume of cecum contents (~3–5 mL). This ensured that we observed
at least two peaks for repressilator signals in individual channels (YFP or CFP)
for a majority of the cells, which is necessary to calculate the period of
oscillation. To minimize phototoxicity the frequency of imaging was kept at
6 min/frame. This gives about 4–5 snapshots per generation time, which is enough
to get a good estimate of growth rate and also a smooth intensity time-series. For E. coli PAS715 experiments imaging
occurred at 10 min/frame. Images were acquired using a Nikon Ti inverted microscope equipped
with a temperature-controlled incubator (OKO lab), a sCMOS camera (ANDOR), a 40X
Plan Apo air objective (NA 0.95, Nikon), an automated xy-stage (Nikon) and light
engine LED excitation source (Lumencor SpectraX). All experiments were performed
at 37 °C. Microscope control was done with Nikon Elements software. We acquired
time-lapse data from 40 fields of view, which allows us to track approximately
2000 cells simultaneously. The acquired data were analyzed using a hybrid
analysis platform written in the Paulsson lab. In brief, images were segmented
using a custom-designed FIJI plugin and then the extracted data were further
processed to track cells in a custom-designed MATLAB script. Time-series of
cell-size data calculated from the segmented images was used to compute
generation times. The time-series of YFP channel intensity was used to calculate
the period of repressilator in the cecum content. Figure generation Figures were generated through Adobe Illustrator CC2018 and CC2019,
Adobe InDesign CC2018 and CC2019, Prism v6-7 (Graphpad), and MATLAB versions
R2017a-2018a (Mathworks). Many figures utilize color palettes based on research
by Cynthia Brewer [55] .